Fibroblast growth factor signalling controls nervous system patterning and pigment cell formation inCiona intestinalis During the development of the central nervous system (CNS), combinations of transcription factors and signalling molecules orchestrate patterning, specification and differentiation of neural cell types. In vertebrates, three types of melanin-containing pigment cells, exert a variety of functional roles including visual perception. Here we analysed the mechanisms underlying pigment cell specification within the CNS of a simple chordate, the ascidian Ciona intestinalis . Ciona tadpole larvae exhibit a basic chordate body plan characterized by a small number of neural cells. We employed lineage-specific transcription profiling to characterize the expression of genes downstream of fibroblast growth factor signalling, which govern pigment cell formation. We demonstrate that FGF signalling sequentially imposes a pigment cell identity at the expense of anterior neural fates. We identify FGF-dependent and pigment cell-specific factors, including the small GTPase, Rab32/38 and demonstrated its requirement for the pigmentation of larval sensory organs. Distinct combinations of transcription factors (TFs) and signalling molecules define the complex gene regulatory networks that control patterning and commitment of different cell types. In vertebrate embryos, pigment-producing cells originate from the closing neuroepithelium: Retinal pigment epithelium (RPE) of the eye and pigment cells of the pineal organ arising from the neural tube; melanocytes of the inner ear, skin, derive from a population of cells migrating from the neural plate border (neural crest) [1] . Despite their different embryological origins, all vertebrate pigment cells share some basic characteristics: melanin pigments are synthesized and stored in melanosomes involving tyrosinase (tyr) and tyr-related enzymes. Melanosomes are tissue-specific lysosome-related organelles distributed in the cell by a regulated vesicular trafficking system, which requires several Rab-type small GTPases and their regulators [2] , [3] . The development of vertebrate RPE and neural retina involves complex interplays among cell-signalling and cell-intrinsic factors: Wnt, bone morphogenetic proteins and fibroblast growth factors (FGFs) [4] , [5] . Among the documented roles for signalling pathways in the formation of the vertebrate visual system, FGF is required to induce neural retina progenitors at the expense of RPE formation [4] , [6] . Nevertheless, understanding the molecular impacts of cell-extrinsic components on cell-specific determinants in the developing of the retina remains a challenging task. Ascidians belonging to the chordate group represent an attractive model system to investigate the generation of cell diversity in the central nervous system (CNS). Despite their highly divergent adult body plan and genomic architecture, phylogenomic analyses indicated that tunicates are the closest living relatives of the vertebrates [7] . The reduced genetic redundancy found in the compact tunicate genome facilitates functional analyses of homologous TFs and signalling molecules in the context of the typical chordate body plan of embryos and larvae. The ascidian Ciona intestinalis emerged as an experimental system of choice due to their simple embryos, rapid development and straightforward transgenesis methods [8] , [9] . Because the ascidian cell lineages and fate maps are well characterized [10] , the identification of neural precursors starting from early fate restriction facilitates the study of progressive cell fate specification in individual precursors through each division. Thus, it is possible to investigate the cellular and molecular mechanisms underlying fate specification with single-cell resolution during the development of chordate CNS. The Ciona tadpole larva offers the advantage of a typical chordate body plan with a simple brain [11] . The anterior sensory vesicle contains two distinct pigment cell containing sensory organs: the geotactic otolith, a single cell containing a melanin granule [12] and the photosensitive ocellus, composed of 30 photoreceptor cells, three lens cells and one cup-shaped pigment cell [13] Ascidian pigment cells express the melanogenic enzyme-coding genes tyrosinase ( tyr ) and tyr -related protein [14] , in a fashion similar to the vertebrate pigment cells [15] . Moreover, Ciona cephalic melanocyte lineage expresses neural plate border and neural crest specification genes, like Id , Snail , Ets and FoxD and the signalling events and regulatory inputs leading to ascidian ocellus formation are similar to those involved in vertebrate neural crest lineage specification, including canonical Wnt and FoxD-mediated repression of Mitf [16] . We recently showed that the FGF/MAPK/Ets pathway is responsible for pigmented cell precursor specification, starting from the late gastrula stage, by rendering their progenies competent to respond to a Wnt signal [17] . However, the FGF signalling downstream targets involved in the regulatory architecture of pigment cell lineage formation remain uncharacterized. Here, we employed a transcriptomic approach by exploiting targeted interference of the FGF signalling coupled with the enrichment of cells of interest by fluorescence-activated cell sorting (FACS) to obtain pigment cell lineage-specific transcription profiles. By using ‘reverse engineering’ methods, we created a pigment lineage-specific co-regulated network to identify key effectors for pigmentation. By characterizing the transcriptional response to FGF signalling in the pigment cell lineage, we identified molecular mechanisms underlying anterior–posterior patterning of Ciona CNS and identified novel regulators of pigment cell specification and differentiation. FGF dependent Pigment cell precursors transcription profiles In ascidians, the pigment cells of the otolith and ocellus arise from the paired a8.25 blastomeres [10] , [18] . During gastrulation, these blastomeres divide and form a9.49 and a9.50 cell pairs: the a9.50s (located in the row IV of the neural plate) are progenitor cells of the anterior brain, while the a9.49s (located in the row III) become fate restricted as pigment cell precursors (PCPs) ( Fig. 1a ) [17] . At the mid-neurula stage (stage 15; Four-dimensional Ascidian Body Atlas [19] ), bilateral PCPs divide, forming two cell pairs (a10.98s and a10.97s, Fig. 1b,c ). Taking advantage of the stability and brightness of 2xGFP reporter driven by tyrp1/2a enhancer ( tyrp1/2a >2xGFP), we observed that a10.97/a10.98s, previously described as a postmitotic pigment cell precursor [20] , undergo an additional division forming eight cells (four on each side) ( Fig. 1d ). An extra a10.97 cell division was also suggested in a note added in proof of Abitua et al . [16] and recently confirmed in Haupaix et al. (see note added in proof.). 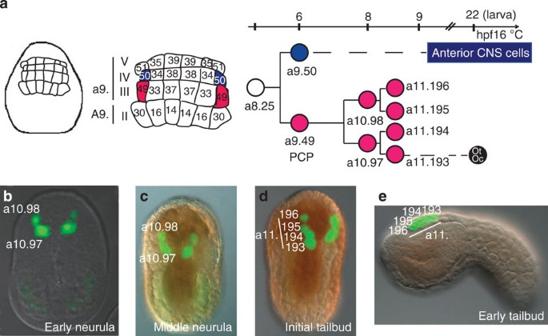Figure 1: TheCionaneural plate and cell lineage of the PCPs. (a, left) Schematic representations of the bilaterally symmetrical embryo at the late gastrula stage with higher magnification of neural plate scheme from row II to V; the PCP a9.49 cell pairs are indicated in pink while their sister cells (a9.50s) are in blue. (a, right) Pigmented cell lineage, right side is shown: letters and numbers indicate cell names according to the referred cell lineages. The approximate timeline applies to the diagrams and lineage tree (hpf, hours post fertilization). Cells with the same colours are derived from a single cell at the late gastrula stage; only the a11.193 cell pair (in black) differentiates into pigment cells at larval stage. Merged bright field/fluorescent images of embryos from early neurula (b) to tailbud stages (c–e) electroporated with ptyrp1/2a>2xGFP cells expressing the GFP (green) and correspond to pigment cell lineage-specific expression. Oc, ocellus, ot, otolith. Figure 1: The Ciona neural plate and cell lineage of the PCPs. ( a , left) Schematic representations of the bilaterally symmetrical embryo at the late gastrula stage with higher magnification of neural plate scheme from row II to V; the PCP a9.49 cell pairs are indicated in pink while their sister cells (a9.50s) are in blue. ( a , right) Pigmented cell lineage, right side is shown: letters and numbers indicate cell names according to the referred cell lineages. The approximate timeline applies to the diagrams and lineage tree (hpf, hours post fertilization). Cells with the same colours are derived from a single cell at the late gastrula stage; only the a11.193 cell pair (in black) differentiates into pigment cells at larval stage. Merged bright field/fluorescent images of embryos from early neurula ( b ) to tailbud stages ( c – e ) electroporated with ptyrp1/2a>2xGFP cells expressing the GFP (green) and correspond to pigment cell lineage-specific expression. Oc, ocellus, ot, otolith. Full size image Following cell nomenclature previously described in Cole and Meinertzhagen [20] , we referred to these cells as a11.196 and a11.195 for the two anterior cells as a11.194 and a11.193 for the two posterior ones ( Fig. 1d,e ). Among the tyrp1/2a + cells, only the two most posterior become otolith and ocellus pigment cells [17] . We recently demonstrated that FGF signalling induces PCP’s formation [17] . We perturbed the endogenous FGF signalling by using a dominant-negative form of the unique Ci-FGF receptor (FGFR DN ) and a constitutively active form of Ci-Ets1/2 (Ets:Vp16) (ref. 21 ), a transcriptional effector of FGF/MAP kinase cascade [22] that is predominantly expressed in all the row III cells, including PCPs, at late gastrula stage [17] . Targeted expression of FGFR DN or Ets:Vp16 in PCPs caused larvae to either lack pigment cells or form extra pigment cells in the sensory vesicle, respectively [17] ( Fig. 2a–c ). 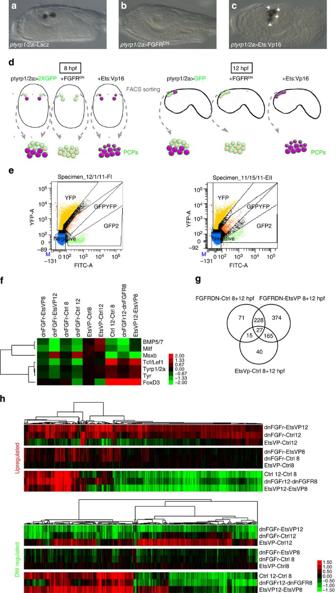Figure 2: Pigment cell lineage-specific transcription profile. Phenotype of larvae electroporated with ptyrp1/2a>LacZ (a), ptyrp1/2a>FGFRDN(b), ptyrp1/2a>Ets:Vp16 (c) observed with transmitted light. Lateral view, anterior is on the left. (d) Schematic representation illustrating the microarray experimental design in two developmental stages, neurula (8 hpf) and tailbud stage (12 hpf); PCPs-lineage cells for microarray analysis were sorted based on their GFP fluorescence.tyrp1/2aenhancer drives target expression of FGFRDNor Ets:Vp16 in PCPs; FGFRDNand Ets:Vp16 conditions mimic regression (light pink) or expansion (dark pink) of the pigmented cells, respectively; (e) FACS plots: ptyrp1/2a>2xGFP (8 hpf, right), ptyrp1/2a>GFP (12 hpf, left) and pMyoD>YFP-expressing cells are distinguished by their green or yellow fluorescence, respectively (hpf, hours post fertilization). The GFP-only quadrant (GFP2) was used to sort PCPs. (f) Hierarchical clustering and heat map: training data set expression values (log2FC) consisting of known PCP markers (Ci-tyr,Ci-tyrp1/2a,Ci-Tcf/Lef,Ci-Mitf,Ci-bmp5/7,Ci-msxbandCi-FoxD). Clustering was performed taking in account all three conditions (control, FGFRDN, Ets:Vp16) at the two developmental stages (8 and 12 hpf). Expression levels are colour coded as represented by the colour range below. (g) Identification of 912 probe sets differentially expressed when comparing the two perturbated conditions with each other and with control samples (FGFRDNversus Control, Ets:Vp16 versus Control and FGFRDNversus Ets:Vp16) at 8 and 12 hpf (for more details on transcript selection, see the text); (h) Log2FC of 912 probe sets showing an increased (upregulated) or decreased (downregulated) expressions when FGFRDNis compared with control or Ets:Vp16 conditions. Colours indicate fold change in pairwise comparisons, for example, dnFGFr-EtsVp 12, means differential expression in ptyrp1/2a>FGFRDNcompared with ptyrp1/2a>Ets:VP16 samples sorted at 12 hpf; red indicate upregulation, green downregulation, respectively. See alsoSupplementary Fig. 1. Figure 2: Pigment cell lineage-specific transcription profile. Phenotype of larvae electroporated with ptyrp1/2a>LacZ ( a ), ptyrp1/2a>FGFR DN ( b ), ptyrp1/2a>Ets:Vp16 ( c ) observed with transmitted light. Lateral view, anterior is on the left. ( d ) Schematic representation illustrating the microarray experimental design in two developmental stages, neurula (8 hpf) and tailbud stage (12 hpf); PCPs-lineage cells for microarray analysis were sorted based on their GFP fluorescence. tyrp1/2a enhancer drives target expression of FGFR DN or Ets:Vp16 in PCPs; FGFR DN and Ets:Vp16 conditions mimic regression (light pink) or expansion (dark pink) of the pigmented cells, respectively; ( e ) FACS plots: ptyrp1/2a>2xGFP (8 hpf, right), ptyrp1/2a>GFP (12 hpf, left) and pMyoD>YFP-expressing cells are distinguished by their green or yellow fluorescence, respectively (hpf, hours post fertilization). The GFP-only quadrant (GFP2) was used to sort PCPs. ( f ) Hierarchical clustering and heat map: training data set expression values (log 2 FC) consisting of known PCP markers ( Ci-tyr , Ci-tyrp1/2a , Ci-Tcf/Lef , Ci-Mitf , Ci-bmp5/7 , Ci-msxb and Ci-FoxD ). Clustering was performed taking in account all three conditions (control, FGFR DN , Ets:Vp16) at the two developmental stages (8 and 12 hpf). Expression levels are colour coded as represented by the colour range below. ( g ) Identification of 912 probe sets differentially expressed when comparing the two perturbated conditions with each other and with control samples (FGFR DN versus Control, Ets:Vp16 versus Control and FGFR DN versus Ets:Vp16) at 8 and 12 hpf (for more details on transcript selection, see the text); ( h ) Log 2 FC of 912 probe sets showing an increased (upregulated) or decreased (downregulated) expressions when FGFR DN is compared with control or Ets:Vp16 conditions. Colours indicate fold change in pairwise comparisons, for example, dnFGFr-EtsVp 12, means differential expression in ptyrp1/2a>FGFR DN compared with ptyrp1/2a>Ets:VP16 samples sorted at 12 hpf; red indicate upregulation, green downregulation, respectively. See also Supplementary Fig. 1 . Full size image Here, we employed FACS and microarray analyses to obtain PCP lineage-specific transcription profiles and identify FGF downstream genes responsible for Ciona PCPs formation. We used the same tyrp1/2a enhancer [14] to express FGFR DN , Ets:VP16 and green fluorescent protein (GFP) and FAC-sort a9.49 cells and their progeny as GFP + cells ( Fig. 2d,e ). To avoid a contamination by mesenchymal cells where Ciona enhancers are often ectopically activated, we co-electroporated the MyoD905>YFP (yellow fluorescent protein) construct and counter-selected YFP + cells as previously described [23] , [24] ( Fig. 2e ). To gain insight into the temporal deployment of the FGF signalling regulatory network, we examined the transcription profiles of PCPs isolated at two developmental stages: 8 hpf at ~16 °C (neurula stage) corresponding to early FGF-mediated induction, and 12 hpf at ~18 °C tailbud(TB) stage, where PCPs are already fate restricted as pigment cells ( Fig. 2d ). The entire data set of 24 microarrays was analysed to identify new candidates involved in the PCP-specific FGF/MAPK/Ets-dependent regulatory network ( Supplementary Fig. 1 ). Correlation analyses of normalized expression values among replicates indicated that microarray experiments were highly reproducible ( Supplementary Fig. 1 ). To explore the expression data set, we reasoned that pigment cell-specific genes should be downregulated upon misexpression of FGFR DN and/or upregulated by Ets:Vp16 compared with controls ( Fig. 2h ), given that FGFR DN blocks pigmentation while Ets:Vp16 causes the formation of supernumerary pigment cells in the PCP lineage [17] ( Fig. 2a–c ). The quadruplicate experiments were used to compute adjusted P values, corrected for multiple testing errors. We first examined the expression values for a training data set consisting of known PCP markers, including Ci-tyr , Ci-tyrp1/2a [14] , Ci-Tcf/Lef [17] , Ci-Mitf , Ci -Bmp5/7 and Ci-msxb [25] ( Fig. 2f ). When comparing their expression levels in FGFR DN versus Ets:Vp16 12hpf samples, the melanogenic genes, Ci-tyr , Ci-tyrp1/2a , the direct FGF downstream gene and transcriptional effector of canonical Wnt signalling Ci-Tcf/Lef as well as known factors involved in pigment cell formation, Ci-Mitf and Ci-Bmp5/7 , were strongly downregulated ( Fig. 2f ). Ci-Mitf and Ci-Bmp5/7 expressions decrease between 8 and 12 hpf. This is in agreement with their early expression in the pigment cell lineage ( Supplementary Fig. 2a,b ; ref. 16 ) and is probably related to their early regulatory function. PCP expression of the transcription regulator Ci-msxb decreased over time, while FGFR DN increased its expression at 12 hpf. These observations are consistent with in situ hybridization (ISH) assays revealing that Ci-msxb is expressed in the 8 hpf neural plate, including the PCPs, while it is excluded from most of the a9.49 derivatives in 12 hpf tailbud embryos, except for the most anterior a11.195s and a11.196s, as demonstrated by the co-localization with Ci-tyrp1/2a ( Supplementary Fig. 2c,d ). According to the extra cell division observed for pigment cell lineage, tyrp1/2a transcripts accumulated preferentially in a10.97s rather than a10.98s retaining a stronger expression in a10.97 progeny (a11.193s/a11.94s) than a10.98s derivatives (a11.195s/a11.96s) that maintains only a residual amount of tyrp1 /2a RNAs. Thus, our microarray data recapitulated distinct tissue-specific expression dynamics: Ci-msxb is downregulated within the PCP lineage between 8 and 12 hpf, but it is maintained in surrounding non-pigmented CNS cells and therefore ectopically expressed in 12 hpf PCPs on inhibition of FGF signalling. Taken together, these observations indicate that our microarray data set efficiently captured known PCP gene activities and probably offers an appropriate representation of pigment cell-specific transcription profiles. FGF signalling opposes the anterior neural plate fate in PCPs To consider all the experimental conditions used for microarray analysis, we focused on 912 probe sets that were differentially expressed when comparing the two perturbated conditions to each other and with control samples (FGFR DN versus Control, Ets:Vp16 versus Control and FGFR DN versus Ets:Vp16) at 8 and 12 hpf ( Fig. 2g ). Since FGF inhibition reprograms PCPs into non-pigmented cells, we first ought to characterize the transcription profiles underlying this fate change. We reasoned that genes upregulated upon FGF inhibition reflect the CNS fate alternative to PCP. We found 461 probe sets corresponding to 264 unique ‘FGF-inhibited’ genes ( Fig. 2h ). Most of these genes were also more highly expressed at 8 than 12 hpf ( Fig. 2h ). Considering that CNS regionalization and cell fate specification take place in early development, we expected that genes involved in these processes would be more highly expressed at early stages. Thus, we reasoned that early ‘FGF-inhibited’ genes would reflect the respecification of a9.49 lineage and illuminate the role of FGF signalling in CNS patterning and early PCP specification. Among the upregulated genes, that is, more highly expressed in FGFR DN samples and/or decreased expression in Ets:Vp16 in comparison with control samples, we first focused on Ci-Six3/6 , a known transcription factor-coding gene expressed in anterior neural domains throughout the animal kingdom [26] , [27] . In Ciona , it is expressed at late gastrula stage in the neural plate IV row of cells, including in daughters of the a9.50 cells ( Fig. 3a ), the sisters of a9.49 PCP precursors located on neural plate III row ( Fig. 1a,b and in Moret et al . [26] ). Double whole-mount ISH (WMISH) demonstrated that Ci-Six3/6 is expressed in a territory that is adjacent but not overlapping with the domain of Ci-tyrp1/2a expression at the neurula to tailbud stages ( Fig. 3a,b ). 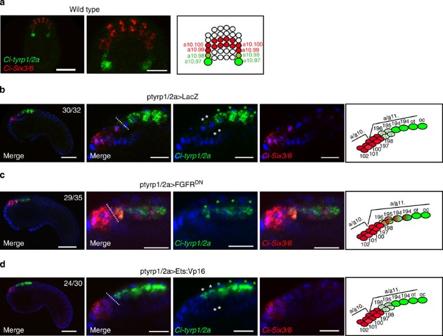Figure 3: FGF signalling imposes anterior neural plate fate in PCPs. Double fluorescent whole-mountin situhybridization (WMISH) with tyramide staining forCi-Six3/6(red) andCi-tyrp1/2a(green) at neurula stage ofCionawild-type embryo (a) and at tailbud stage ofCionaelectroporated embryos with ptyrp1/2a>LacZ (b), ptyrp1/2a>FGFRDN(c) and ptyrp1/2a>Ets:Vp16 (d) plasmids. Zoom on the expression domains, dashed line indicate the border amongCi-Six3/6andCi-tyrp1/2a-positive cells. Embryos showing separate channels fortyrp1/2a(green) that marks a10.97 derivatives (green asterisks) and very faintly a10.98s progenies (white asterisks) andSix3/6(red) expression. On the right, schematic illustration ofCionaneural plate and neural tube cells at tailbud stage showingCi-Six3/6(red) andCi-tyrp1/2a(green) expressing cells, adapted from Cole and Meinertzhagen, 2004. (a)Vegetal view, anterior is on the top; (b–d) lateral view, anterior is on the left. Scale bar, 50 μm; for zoomed embryos, scale bar, 20 μm; nuclear staining by DAPI (blue). Number (n) of embryos showing the observed phenotype out of the total counted embryos, referred to one experiment that was repeated at least three times. See alsoSupplementary Fig. 3. Figure 3: FGF signalling imposes anterior neural plate fate in PCPs. Double fluorescent whole-mount in situ hybridization (WMISH) with tyramide staining for Ci-Six3/6 (red) and Ci-tyrp1/2a (green) at neurula stage of Ciona wild-type embryo ( a ) and at tailbud stage of Ciona electroporated embryos with ptyrp1/2a>LacZ ( b ), ptyrp1/2a>FGFR DN ( c ) and ptyrp1/2a>Ets:Vp16 ( d ) plasmids. Zoom on the expression domains, dashed line indicate the border among Ci-Six3/6 and Ci-tyrp1/2a- positive cells. Embryos showing separate channels for tyrp1/2a (green) that marks a10.97 derivatives (green asterisks) and very faintly a10.98s progenies (white asterisks) and Six3/6 (red) expression. On the right, schematic illustration of Ciona neural plate and neural tube cells at tailbud stage showing Ci-Six3/6 (red) and Ci-tyrp1/2a (green) expressing cells, adapted from Cole and Meinertzhagen, 2004. ( a )Vegetal view, anterior is on the top; ( b – d ) lateral view, anterior is on the left. Scale bar, 50 μm; for zoomed embryos, scale bar, 20 μm; nuclear staining by DAPI (blue). Number (n) of embryos showing the observed phenotype out of the total counted embryos, referred to one experiment that was repeated at least three times. See also Supplementary Fig. 3 . Full size image To mirror microarray experiments, we performed double WMISH using Ci-Six3/6 and Ci-tyrp1/2a probes following FGF perturbations. In Ets:Vp16 electroporated embryos and control samples, we did not detect any change in Ci-Six3/6 expression ( Fig. 3d ), while FGF inhibition caused ectopic Ci-Six3/6 expression in a posterior domain that includes Ci-tyrp1/2a -positive a9.49 derivatives ( Fig. 3c ). These findings recapitulate the microarray data and indicate that FGF signalling normally inhibits Ci-Six3/6 expression in Ci-tyrp1/2a + PCPs. To characterize the FGF regulatory network that generate cell identity in the anterior CNS of the tailbud embryos, we analysed the expression pattern of genes encoding TFs that were significantly upregulated when comparing FGFR DN with Ets:Vp16 in 12 hpf PCPs. Among 21 genes, we selected Ci-Pax3/7 , Ci-Macho-1 , Ci-FoxHa , Ci-msxb and Ci-Pax6 . We included additional genes with published expression profiles in the ANISEED database [28] : Ci-RGR/Nut , Ci-Neurogenin ( Ngn ) and Ci-COE [25] that are widely expressed in the CNS. We then asked whether these genes co-localize with Ci-Six3/6 + anterior neural cells in tailbud embryos. All these genes were expressed in anterior neural domains, overlapping with Ci-Six3/6 ( Supplementary Fig. 3a–i ). According to published neural lineages [20] , this domain located anteriorly to the prospective PCP includes a10.100s, a11.198s and a11.197s, all derived from the a9.50 blastomeres, which already express Ci-Six3/6 in early neurula embryos and are a9.49 sister cells ( Supplementary Fig. 3a ). Our observations that Ci-Six3/6 and other markers of a9.50 derivatives were upregulated by FGFR DN misexpression in the a9.49 lineage indicate that FGF signalling promotes PCP specification in a9.49 derivatives by inhibiting a9.50 specification including Ci-Six3/6 expression, thus specifying different anterior-to-posterior fates within the neural plate. These results indicate that the most posterior Ci-Six3/6 + cells express a unique combination of genes, which are inhibited by FGF signalling in the adjacent PCPs. As further support, we found that anterior CNS markers, as Ci-Pax3/7 , Ci-Pax6 , Ci-COE , are ectopically expressed posteriorly in PCPs domain when FGF signalling is specifically inhibited in these cells ( Supplementary Fig. 4 ). Progressive PCP induction by sequential FGF/MAPK signalling Starting from early gastrulation, the FGF signal is released from the A-nerve cord precursors and induces the a8.25 blastomeres, subsequentially their progenies (a9.49s), as future pigment cells [17] , [18] , [29] . To determine the timing of MAPK activation during PCP divisions in a10.97/a10.98s and in their progeny, we performed immunostaining assays of the dual-phosphorylated (dp) form of ERK1/2 (ref. 29 ). At late gastrula stage, dpERK appears in the a-line neural plate in the row III cells, including a9.49s, but not on the row IV that includes Ci-Six3/6 -expressing cells, as shown in Hudson et al. [29] Later in development, we detected dpERK staining in the a10.97s but not in a10.98s ( Fig. 4a–c ). After the second round of PCP division, dpERK staining remains in a10.97 progenies, appearing stronger in the precursors of otolith and ocellus pigmented cells (a11.193s) than in a11.194s ( Fig. 4d ). These data suggest that the MAPK activation is progressively restricted to the posterior PCPs, the sole to become pigmented at later stage. We next used timed inhibition of MAPK signalling to further test whether sequential induction of FGF signalling corresponds to successive steps in PCP specification. To this aim, we followed PCP division by assaying GFP reporter expression and placed embryos in the pharmacological agent U0126 to block the MEK kinase for 30 min at gastrula (a9.49s), neurula (a10.97s/a10.98s) and early tailbud (a11.193s/a11.194s and a11.195s/a11.196s) stages. We then observed the presence of pigmented cells in the larval sensory vesicle. As already demonstrated, the resulting larvae completely lacked pigment cells when embryos were treated at gastrula stage [17] . We found that when embryos were treated at neurula and early tailbud stages, larvae deprived of pigment cells decreased ( Fig. 5a ) while a little effect was observed when embryos were placed in UO126 after the final cell division (a11.193s) of pigment cell lineage. These data are in according to the differential activation of ERK1/2 in PCPs that appeared stronger in the a10.97s and their progenies than the other PCP cells. 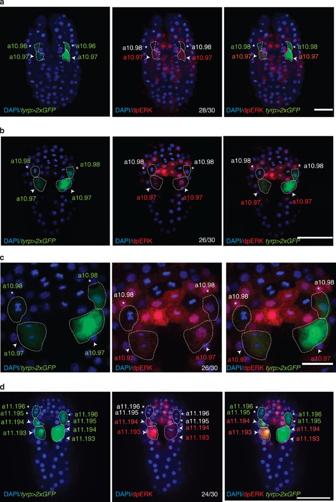Figure 4: Sequential induction mediated gradually by FGF/MAPK/ERK on PCPs. Activation of ERK1/2 visualized by dpERK1/2 antibody staining.Cionaembryos were electroporated with ptyrp1/2a>2xGFP and stained using anti-GFP antibody (green) to label the PCPs from early neurula (a) (a10.97s and a10.98s), late neurula (b,c) (a10.97s and a10.98s in division) to early tailbud stage (d) (a11.194s, a11.195s and a11.196s). Note that at early and late neurula stages, nuclear dpERK is detected in the a10.97s and their progenies but not in a10.98s. (a,b,d) Scale bar, 50 μm; (c) scale bar, 20 μm; nuclear staining is visualized by DAPI (blue). White asterisks and arrowhead indicate a10.98s and a10.97s and their cell progenies, respectively. Number of embryos showing dpERK1/2 staining out of the total embryos scored. Each experiment was repeated at least three times. Figure 4: Sequential induction mediated gradually by FGF/MAPK/ERK on PCPs. Activation of ERK1/2 visualized by dpERK1/2 antibody staining. Ciona embryos were electroporated with ptyrp1/2a>2xGFP and stained using anti-GFP antibody (green) to label the PCPs from early neurula ( a ) (a10.97s and a10.98s), late neurula ( b , c ) (a10.97s and a10.98s in division) to early tailbud stage ( d ) (a11.194s, a11.195s and a11.196s). Note that at early and late neurula stages, nuclear dpERK is detected in the a10.97s and their progenies but not in a10.98s. ( a , b , d ) Scale bar, 50 μm; ( c ) scale bar, 20 μm; nuclear staining is visualized by DAPI (blue). White asterisks and arrowhead indicate a10.98s and a10.97s and their cell progenies, respectively. Number of embryos showing dpERK1/2 staining out of the total embryos scored. Each experiment was repeated at least three times. 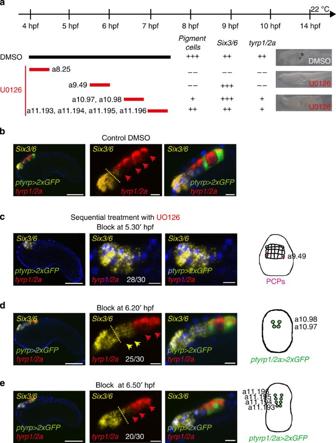Figure 5: Sequential FGF-MAPK signalling is required to inhibit expression of anterior CNS markers in PCP territories. (a) Summary model of the timed inhibition of MAPK signalling using UO126 treatment. Wild-typein vitrofertilized embryos were treated with U0126 at the gastrula, neurula and early tailbud stages for 30 min at room temperature.Cionaembryos were electroporated with ptyrp1/2a>2xGFP to label the PCPs and stained with anti-GFP (green) antibody. (b) Control embryos incubated with dimethylsulphoxide showingCi-Six3/6(yellow) andCi-tyrp1/2a(red) expression at tailbud stage. Dashed line indicates the border amongCi-Six3/6andCi-tyrp1/2aendogenous expression pattern. (c) Sequential treatment with UO126 at 5h 30′ (a9.49 PCPs), at 6h 20′ (d) (a10.97s and a10.98s) and 6h 50′ (e) (a11.193s, a11.194s, a11.195s and a11.196s) showing alteration inCi-tyrp1/2a(red) andCi-Six3/6 (yellow) expression in PCPs. Lateral view, anterior towards the left. Scale bar, 50 μm; scale bar, 20 μm, for zoomed embryos. Number (n) of embryos showing the observed phenotype out of the total counted embryos, referred to one experiment that was repeated at least three times. Nuclear staining is visualized by DAPI (blue). Full size image Figure 5: Sequential FGF-MAPK signalling is required to inhibit expression of anterior CNS markers in PCP territories. ( a ) Summary model of the timed inhibition of MAPK signalling using UO126 treatment. Wild-type in vitro fertilized embryos were treated with U0126 at the gastrula, neurula and early tailbud stages for 30 min at room temperature. Ciona embryos were electroporated with ptyrp1/2a>2xGFP to label the PCPs and stained with anti-GFP (green) antibody. ( b ) Control embryos incubated with dimethylsulphoxide showing Ci-Six3/6 (yellow) and Ci-tyrp1/2a (red) expression at tailbud stage. Dashed line indicates the border among Ci-Six3/6 and Ci-tyrp1/2a endogenous expression pattern. ( c ) Sequential treatment with UO126 at 5h 30′ (a9.49 PCPs), at 6h 20′ ( d ) (a10.97s and a10.98s) and 6h 50′ ( e ) (a11.193s, a11.194s, a11.195s and a11.196s) showing alteration in Ci-tyrp1/2a (red) and Ci-Six3/ 6 (yellow) expression in PCPs. Lateral view, anterior towards the left. Scale bar, 50 μm; scale bar, 20 μm, for zoomed embryos. Number ( n ) of embryos showing the observed phenotype out of the total counted embryos, referred to one experiment that was repeated at least three times. Nuclear staining is visualized by DAPI (blue). Full size image We then examined Ci-Six3/6 + and Ci-tyrp1/2a + cells at tailbud stage following Ci-Six3/6 and Ci-tyrp1/2a transcripts, together with GFP expression driven by tyrp1/2a enhancer ( ptyrp1/2a >2xGFP) as pigment cell lineage marker ( Fig. 5b ). Upon treatment at 5h30′ (a9.49s), Ci-tyrp1/2a expression is lost in PCPs ( Fig. 5c ) whereas it is strongly reduced when embryos were treated at the neurula stage (10.97s/a10.98s) ( Fig. 5d ) and appeared almost normal when the drug was applied at early tailbud stage (a11.193s/a11.194s) ( Fig. 5e ); by contrast, Ci-Six3/6 detection is always expanded posteriorly in the CNS, although to a lesser extent upon later treatments. The results obtained with successive U0126 treatments show that MAPK activity is necessary at each sequential PCP division (a9.49 and a10.97/a10.98 division) to direct PCPs through their final fate from gastrula to tailbud stage and became less effective when PCP became post mitotic (a11.193s/a11.194s). Expression of new marker genes for pigment cell lineage We next ought to identify novel genes expressed in the PCP downstream of FGF signalling. Since FGF signalling is implicated in Ciona pigment cell formation [17] , we reasoned candidate PCP-specific FGF targets should be either downregulated by FGFR DN and/or upregulated by Ets:Vp16 at 8 or 12 hpf and identified 451 probe sets matched to 207 unique annotated genes ( Fig. 2h ). Gene ontology (GO) terms analyses indicated that the pool of candidate PCP-specific FGF targets are enriched for genes involved in melanization with overrepresented processes such as ‘pigmentation’, ‘pigment binding’, ‘melanocyte differentiation’ and ‘eye pigment biosynthetic process’ thus confirming the validity of our approach and its potential for the discovery of novel PCP-specific candidates involved in melanization that are under the control of FGF signalling ( Supplementary Table 1 ). To gain insights into the FGF-dependent regulatory network controlling pigment cell formation, we analysed the expression values of candidate PCP genes encoding TFs and signalling molecules. We identified 20 regulatory genes that might contribute to PCP fate specification ( Supplementary Fig. 5 ). We identified the conserved FGF/MAPK pathway components MAPKK7, Dusp1.2.4.5, Dusp6.9 and ELK1/3 (ref. 31 ), the BMP-family ligands Bmp5/7, Bmp2/4 (ref. 31 ) and Wnt signalling molecules such as the downstream effector Tcf/Lef, Wnt14/15, Frizzled receptor (Orphan Fz-a), the Wnt-co-receptors Lrp4 and Lrp1b and the secreted Wnt antagonist Dickkopf1 (Dkk1) (ref. 32 ). Interestingly, genes encoding the secreted BMP antagonists, Ci-noggin [33] as well as Ci-BMPER , a BMP-binding antagonist [34] , were upregulated in FGFR DN compared with Ets:Vp16 samples. Taken together, these data suggest that the FGF/MAPK pathway potentiates BMP signalling during PCP fate specification and provides further insight into the interaction between FGF and Wnt that we previously uncovered [17] . To find new PCP-specific markers, we selected 30 genes among the downregulated genes identified from the pairwise comparisons (FGFR DN versus Ets:Vp16 and FGFR DN versus control) for subsequent ISH analyses. We obtained a specific CNS staining for 14 of the PCP candidates. Among these, six genes ( Ci-Lrp4, Ci-Bzrap1, Ci-Casz1, Ci-Mad/mnt, Ci-Slc45a2, Ci-Piwi ) showing defined PCP expression were selected for further analysis ( Fig. 6a–g ). Double WMISH using the pigment cell marker, Ci-tyrp1/2a [14] , was performed to ascertain PCP-specific expression ( Fig. 6 ). Detailed analysis of the expression domain showed that some genes are expressed in all the eight a9.49-derived cells ( Ci-Mad/Mnt , Ci-Piwi ), while Ci-Casz1 is localized in the posterior six cells; others are exclusively expressed in the posterior two presumptive pigment cells ( Ci-Bzrap1 , Ci-Slc45a2 , Ci-Lrp4 ) ( Fig. 6 ). Furthermore, in situ assays on embryos where FGF signalling was perturbed confirmed that the expression of some candidates ( Ci-Casz1 , Ci-Slc45a2 and Ci-Bzrap1 ) depends upon proper FGF signalling in PCPs ( Fig. 7 ). Thus, our results reveal that each PCP lineage cell at the dorsal midline of the tailbud stage exhibits a unique combination of transcripts. These combinations constitute specific molecular signatures that define individual cell identities in the dorsal CNS. 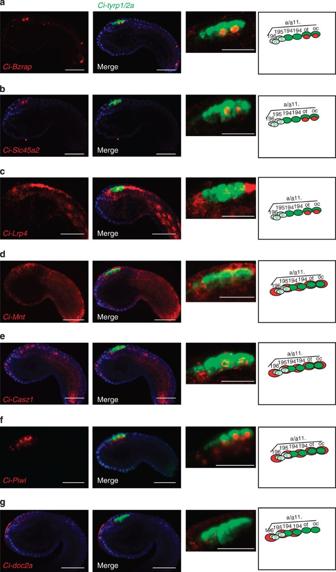Figure 6: Expression ofCionacandidate PCP genes. Expression pattern at tailbud stage of PCP candidate genes (red):Ci-bzrap,(a),Ci-Slc45a2(b),Ci-Lrp4(c),Ci-Mnt(d),Ci-Casz1(e),Ci-Piwi(f) andCi-doc2a(g); co-localization (merge) of these PCP markers withCi-tyrp1/2a(green),higher magnification on the right. Schematic representation of a9.49-derived cells in the neural tube ofCionatailbud stage showingCi-tyrp1/2a+cells (green) and PCP candidates expressing cells (red), adapted from Cole and Meinertzhagen, 2004.tyrp1/2atranscripts are accumulated mostly in a10.97 progeny (a11.193s/a11.94s, green) than a10.98s derivatives (a11.195s/a11.96s, light green) that maintains only a residual amount oftyrp1/2aRNAs. Lateral view, anterior is on the left. Scale bar, 50 μm; scale bar, 20 μm for zoomed embryo; nuclear staining by DAPI (blue). Number of embryos scored was higher than 30; each experiment was repeated at least two times. Figure 6: Expression of Ciona candidate PCP genes. Expression pattern at tailbud stage of PCP candidate genes (red): Ci-bzrap ,( a ), Ci-Slc45a2 ( b ), Ci-Lrp4 ( c ), Ci-Mnt ( d ), Ci-Casz1 ( e ), Ci-Piwi ( f ) and Ci-doc2a ( g ); co-localization (merge) of these PCP markers with Ci-tyrp1/2a (green),higher magnification on the right. Schematic representation of a9.49-derived cells in the neural tube of Ciona tailbud stage showing Ci-tyrp1/2a + cells (green) and PCP candidates expressing cells (red), adapted from Cole and Meinertzhagen, 2004. tyrp1/2a transcripts are accumulated mostly in a10.97 progeny (a11.193s/a11.94s, green) than a10.98s derivatives (a11.195s/a11.96s, light green) that maintains only a residual amount of tyrp1/2a RNAs. Lateral view, anterior is on the left. Scale bar, 50 μm; scale bar, 20 μm for zoomed embryo; nuclear staining by DAPI (blue). Number of embryos scored was higher than 30; each experiment was repeated at least two times. 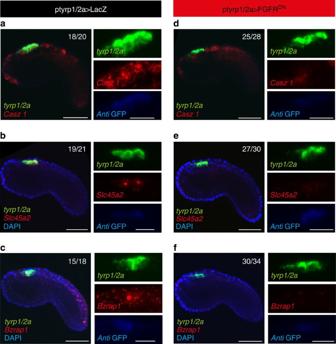Figure 7: FGF signalling controls the expression of new PCP marker genes. Double fluorescent WMISH ofCi-Casz1,Ci-Slc45a2andCi-Bzrap1(red) withCi-tyrp1/2a(green) coupled with immunostaining of GFP (light blue, in zoomed embryos). Embryos are electroporated both with ptyrp1/2a>LacZ (a–c) and ptyrp1/2a>FGFRDN(d–f) and ptyrp1/2a>GFP. Lateral view, anterior is on the left. Scale bar, 50 μm; scale bar, 20 μm, for zoomed embryos; nuclear staining by DAPI (blue); number (n) of embryos showing the observed phenotype out of the total counted embryos, referred to one experiment, that was repeated at least three times. Full size image Figure 7: FGF signalling controls the expression of new PCP marker genes. Double fluorescent WMISH of Ci-Casz1 , Ci-Slc45a2 and Ci-Bzrap1 (red) with Ci-tyrp1/2a (green) coupled with immunostaining of GFP (light blue, in zoomed embryos). Embryos are electroporated both with ptyrp1/2a>LacZ ( a – c ) and ptyrp1/2a>FGFR DN ( d – f ) and ptyrp1/2a>GFP. Lateral view, anterior is on the left. Scale bar, 50 μm; scale bar, 20 μm, for zoomed embryos; nuclear staining by DAPI (blue); number ( n ) of embryos showing the observed phenotype out of the total counted embryos, referred to one experiment, that was repeated at least three times. Full size image Ci-Rab32/38 as ‘hub’ gene in Ciona pigment cell formation To identify key effector genes necessary for Ciona PCPs formation and controlled by FGF signalling, we used a ‘reverse engineering’ approach. This method identifies co-regulated genes, that is, genes that are co-expressed across a set of experimental conditions. Co-regulated genes may be a part of the same pathway, regulated by the same transcription factor, and/or part of the same protein complex [35] , [36] . The reverse engineering approach we used is based on computing correlations across pairs of genes from gene expression profiles [35] , [36] . Specifically, we computed the Spearman correlation coefficient (SCC) values for each pair of probe sets across the 24 microarrays to build a network of co-regulated genes for Ciona PCP (Methods). The resulting gene network consists of 4,755,086 significant ( P value <0.01) predicted connections among 30,969 probe sets. To identify groups of candidate FGF target genes in early PCPs, we built a smaller subnetwork ( Fig. 8a ) by selecting only the top 50 differentially expressed genes (when comparing FGFR DN to control samples at 8 hpf) together with their co-regulated genes from the main network (gene neighbours). In a co-regulatory network, most of the genes are connected to few other genes. Nevertheless, it is possible to identify a relatively small number of genes with a large number of neighbours, called hubs [37] , [38] . In the subnetwork comprising early FGF targets, we identified a set of ‘hub genes’ and ranked them according to the number of neighbours ( Supplementary Table 2 ). The top two hub genes were annotated as unknown protein in the Ciona genome, even though for the second one we found a blast homology with mouse C3a anaphylatoxin chemotactic receptor, part of the rhodopsin family of G protein-coupled receptor [39] . The remaining hub genes were the transcription factor Ci-NF001 , the Ras-related protein Ci-Rab32/38 , the Notch co-activator mastermind, Ci-mam and the Melanophilin, Ci-Mlph , a Rab effector involved in melanosome transport along microtubules ( Supplementary Table 2 ). 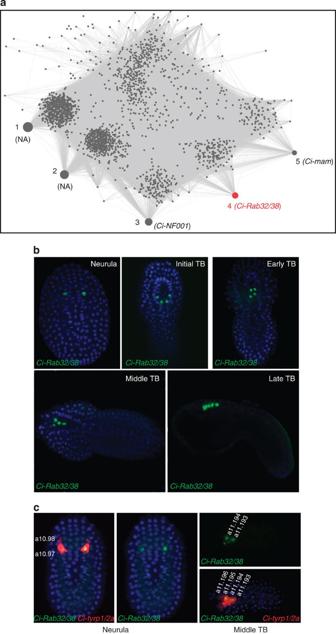Figure 8: Rab-type small GTPases as ‘hub’ gene inCionapigment cell formation. (a) Early PCP-specific subnetwork inferred from the analysis of microarrays. ‘Hub’ genes are represented as grey spots, numbered from 1 to 5, by ranking them according to the number of neighbours.Ci-Rab32/38is evidenced in red. (b)Ci-Rab32/38expression (green) in PCPs duringCionaneurulation: neurula, initial TB, early TB, middle and late TB stages. (c) Double WMISH forCi-Rab32/38(green) andCi-tyrp1/2a(red) from neurula to middle TB stage; nuclear staining by DAPI (blue);n>50 embryos scored for gene expressions. Figure 8: Rab-type small GTPases as ‘hub’ gene in Ciona pigment cell formation. ( a ) Early PCP-specific subnetwork inferred from the analysis of microarrays. ‘Hub’ genes are represented as grey spots, numbered from 1 to 5, by ranking them according to the number of neighbours. Ci-Rab32/38 is evidenced in red. ( b ) Ci-Rab32/38 expression (green) in PCPs during Ciona neurulation: neurula, initial TB, early TB, middle and late TB stages. ( c ) Double WMISH for Ci-Rab32/38 (green) and Ci-tyrp1/2a (red) from neurula to middle TB stage; nuclear staining by DAPI (blue); n >50 embryos scored for gene expressions. Full size image Among the selected hub genes, we focused on the small GTPase Ci-Rab32/38. In vertebrate melanocytes, the two homologous proteins, Rab32 and Rab38, localize to secretory vesicles of the trans -Golgi network where they function redundantly to transport Tyrosinase- and Tyrp1-containing vesicles to the forming melanosomes [40] . The C. intestinalis genome encodes a unique ortholog, Ci-Rab32/38/rab-rp1/ltd ( Ci-Rab32/38 ), showing a significant differential expression when comparing FGFR DN and control at 8 hpf, as confirmed by in situ assays on embryos electroporated with FGFR DN and Ets:Vp16 ( Supplementary Fig. 6a–c ). Starting at the early neurula stage, Ci-Rab32/38 is specifically expressed in two cells that correspond to a10.97s and subsequently in a11.193s and a11.194s at tailbud stage as confirmed by the co-localization with Ci-tyrp1/2a ( Fig. 8b,c ). The specific and early expression of Ci-Rab32/38 in the pigment cell lineage suggested a role in Ciona melanization by regulating vesicle dynamics during pigment cell formation. In keeping with this hypothesis, we observed that a group of genes also implicated in vesicular trafficking and melanosome biogenesis were differentially expressed when FGF signalling is blocked in PCPs between 8 and 12 hpf. This group includes the RabGAP Wdr67, the Rab effector MyRip/Exophilin and other genes involved in exocytosis and vesicle docking (RABEPK, Rab6-interacting kinesin-like protein, MPHOSPH1, ARF3, Doc2a/Rabphilin [41] , which we found expressed in a11.195s and a11.196s PCPs ( Fig. 6g ). These data indicate that FGF signalling regulates Rab GTPases and associated cellular effectors controlling vesicular trafficking during Ciona pigment cell formation. Role of Rab32/38 in Ciona pigment cell formation In vertebrates, mutations in several Rab GTPases and their regulators result in pigmentation defects due to altered platelet and melanosome formation [42] . The chocolate ( cht ) mouse, characterized by a recessive Gly19 to Val mutation, displayed dramatically reduced numbers of melanosomes in adult RPE, in addition to a mild phenotype in skin melanocytes [43] , [44] . Depletion of Rab32 in mildly hypopigmented cht melanocytes severely impairs pigmentation and melanosome morphology indicating that the hypopigmentation defects in cht melanocytes was due to a functional compensation of Rab32 (ref. 40 ). To investigate a possible function of the single Ci-Rab32/38 ortholog gene during Ciona pigmentation process, we first studied the effects of a dominant-negative Ci-Rab32/38 mutant (Rab32/38 G19V ). PCP-targeted expression of Rab32/38 G19V in PCPs using the tyr enhancer [14] altered both otolith and ocellus pigmentation. In more than 70% of larvae, pigmented sensory organs appeared either not or partially melanized ( Fig. 9a ). Considering that mouse Rab38 G19V is unstable because it lacks posttranslational lipid modification that results in premature degradation [40] , we introduced another point mutation in Ci-Rab32/38 G19V altering a second residue in the highly conserved GTPase fold domain (Rab32/38 G19V+T23N ) creating a dominant-negative mutated form (T23N) [45] . Targeted expression of Ci-Rab32/38 G19V+T23N in pigment cell lineage caused a drastic reduction of the proportion of larvae (5%) showing two pigmented cells within the sensory vesicle, with more than 90% of perturbed larvae had alteration in at least one of the two pigmented cells ( Fig. 9a ). To further confirm the role of Ci-Rab32/38, we used short hairpin RNA (shRNA)-mediated RNA interference approach [46] to knock down Ci-Rab32/38 activity and analyze the effect on pigmented cell formation. We used combinations of shRNA constructs targeting two sites in the Ci-Rab32/38 coding region. Double WMISH assays on embryos electroporated with either the U6>shRab32/38-C and -D or U6>shRab32/38-E and -F combination, showed that Ci-Rab32/38 -targeting shRNAs markedly reduced its endogenous expression in PCPs ( Fig. 9c,d ). Expression of two pairs of constructs (U6>shRab32/38-C, -D and U6>shRab32/38-E, -F) resulted in up to 90% larvae showing defective pigment cell melanization ( Fig. 9b ). Taken together, these data indicate that the complete melanization of the pigment cell is thus significantly affected by Ci-Rab32/38 G19V+T23N and Ci-Rab32/38 knockdown experiments, suggesting that proper Ci-Rab32/38 activity has an essential role in pigment cell terminal differentiation. 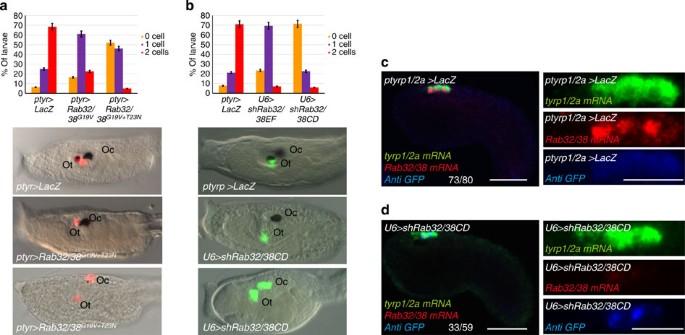Figure 9: Role of Rab32/38 inCionapigment cell biogenesis. Histograms showing the percentage of larvae with two pigment cells (red), one pigment cell (violet) and no pigment cells (orange) after electroporation of dominant-negative forms of Ci-Rab32/38 under control of PCP enhancer (ptyr>Rab32/38G19Vor ptyr>Rab32/38G19V+T36N) (a) or short hairpin inhibiting construct againstCi-Rab32/38mRNA (U6>shRab32/38-C-D and U6>shRab32/38-E-F) (b) compared with control larvae electroporated with ptyr>LacZ.Merged bright field/fluorescent images of transgenic larvae. (c,d) Double fluorescent WMISH was performed to test the ability of U6>shRab32/38 used to knock down the endogenousCi-Rab32/38. The expression ofCi-Rab32/38(red) is compared withCi-tyrp1/2a(green) and with anti-GFP antibody to follow expression of the electroporated constructs. Embryos were electroporated with ptyrp1/2a>GFP plus ptyrp1/2a>LacZ (c) and ptyrp1/2a>GFP plus U6>shRab32/38-C-D (d). U6>shRab32/38-C–D is able to knock down the endogenousCi-Rab32/38transcripts (n=33/59, d) and to induce defects in pigmented sensory organ melanization (a,b), whileCi-tyrp1/2aexpression resulted not affected (c) as compared with the control embryos (n=73/80, c). Anterior to the left; nuclear staining by DAPI (blue). Scale bar, 50 μm; scale bar, 20 μm for zoomed embryos. Within each histogram is the combined number of larvae counted during at least three trials;n>150 embryos scored for transgene expression; error bar, s.e.m.; oc, ocellus, ot, otolith. Figure 9: Role of Rab32/38 in Ciona pigment cell biogenesis. Histograms showing the percentage of larvae with two pigment cells (red), one pigment cell (violet) and no pigment cells (orange) after electroporation of dominant-negative forms of Ci-Rab32/38 under control of PCP enhancer (ptyr>Rab32/38 G19V or ptyr>Rab32/38 G19V+T36N ) ( a ) or short hairpin inhibiting construct against Ci-Rab32/38 mRNA (U6>shRab32/38-C-D and U6>shRab32/38-E-F) ( b ) compared with control larvae electroporated with ptyr>LacZ.Merged bright field/fluorescent images of transgenic larvae. ( c , d ) Double fluorescent WMISH was performed to test the ability of U6>shRab32/38 used to knock down the endogenous Ci-Rab32/38 . The expression of Ci-Rab32/38 (red) is compared with Ci-tyrp1/2a (green) and with anti-GFP antibody to follow expression of the electroporated constructs. Embryos were electroporated with ptyrp1/2a>GFP plus ptyrp1/2a>LacZ ( c ) and ptyrp1/2a>GFP plus U6>shRab32/38-C-D ( d ). U6>shRab32/38-C–D is able to knock down the endogenous Ci-Rab32/38 transcripts ( n =33/59, d) and to induce defects in pigmented sensory organ melanization ( a , b ), while Ci-tyrp1/2a expression resulted not affected ( c ) as compared with the control embryos ( n =73/80, c). Anterior to the left; nuclear staining by DAPI (blue). Scale bar, 50 μm; scale bar, 20 μm for zoomed embryos. Within each histogram is the combined number of larvae counted during at least three trials; n >150 embryos scored for transgene expression; error bar, s.e.m. ; oc, ocellus, ot, otolith. Full size image The combination of cell sorting and transcriptome analyses identified pigment cell lineage candidate genes and provided new insights into the mechanisms of CNS patterning in Ciona . We have shown that FGF signalling functions as successive inputs rather than continuously during induction of PCPs. Sequential FGF inputs influence defined regulatory networks successively controlling early fate specification, the selection of definitive pigment cells within the PCP lineage and the processes that underlie pigment cell differentiation at later stages (summarized in Fig. 10 ). 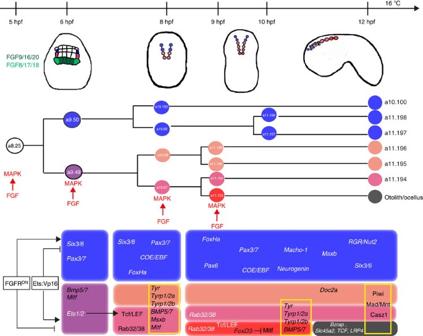Figure 10: FGF/MAPK inputs sequentially govern PCP versus anterior CNS formation. Summary of pigmented cell development within CNS; embryonic stage drawings are indicated below the time line (hpf, hours post fertilization). Black bars connect sister cells. At 6 hpf embryo, the bilateral a9.50s are marked in blue; a9.49 cell pair (in pink) are in close proximity to two sources of FGF signalling molecules, Ci-FGF8/17/18 (light green) and Ci-FGF9/16/20 (dark green) in the underneath row, respectively. Cell lineage scheme indicate one side of the embryo and the colour code of cells remains the same used in the upper drawings. Red arrows indicate FGF/MAPK signalling mediated inductions. a8.25-derived cells with specific gene expression patterns: boxes represent a9.50- and a9.49-derived cells with the same colour code used in the upper drawings. FGFRDN: dominant-negative form of FGF receptor; Ets:Vp16: constitutive active form of Ets1/2. Figure 10: FGF/MAPK inputs sequentially govern PCP versus anterior CNS formation. Summary of pigmented cell development within CNS; embryonic stage drawings are indicated below the time line (hpf, hours post fertilization). Black bars connect sister cells. At 6 hpf embryo, the bilateral a9.50s are marked in blue; a9.49 cell pair (in pink) are in close proximity to two sources of FGF signalling molecules, Ci-FGF8/17/18 (light green) and Ci-FGF9/16/20 (dark green) in the underneath row, respectively. Cell lineage scheme indicate one side of the embryo and the colour code of cells remains the same used in the upper drawings. Red arrows indicate FGF/MAPK signalling mediated inductions. a8.25-derived cells with specific gene expression patterns: boxes represent a9.50- and a9.49-derived cells with the same colour code used in the upper drawings. FGFR DN : dominant-negative form of FGF receptor; Ets:Vp16: constitutive active form of Ets1/2. Full size image Our data elucidate the roles of FGF signalling pathway during differential fate specification and anteroposterior patterning of the Ciona CNS. We show that, in the absence of FGF signalling, PCPs change their fate into anterior CNS cells, as judged by ectopic expression in the a9.49-derived PCPs of genes, which are normally expressed in 9.50s derivatives. According to these observations, we propose that FGF signalling imposes a pigment cell identity at the expense of the anterior CNS cell fate, distinguishing between anterior and posterior identities during the formation of Ciona nervous system. This is reminiscent of the situation in vertebrates, where FGF, together with Wnt signalling act to induce a posterior identity on neural tissue during neurulation [47] , [48] . In chick, FGF derived from the lens ectoderm is necessary to maintain the retina domain in the distal optic vesicle [49] . Moreover in FGF9 mouse mutants, the RPE expands into the presumptive retina suggesting that FGF9 is required to define the boundary between retina and RPE [50] . Our analyses suggest that in Ciona FGF signalling plays an initial role during the induction of pigmented versus anterior CNS cells. This could be related to the position of photoreceptor and pigmented cell precursors on the III row cells of the neural plate, both in close proximity to FGF signalling molecules, Ci-FGF8/17/18 and Ci-FGF9/16/20 (refs 11 , 18 ) ( Fig. 10 ). Although all PCPs have the potential to complete pigment cell differentiation, only the two posterior a11.113s will form the otolith and melanocyte of the ocellus. It is likely that specific transcription profiles impose their cell identity to uniquely defined PCP derivatives. Microarray data identified new candidates involved in Ciona pigment cell formation and showing a distinct gene expression profiles among PCPs (summarized in Fig. 10 ). Although some factors, such as Rab32/38 and Ci-Slc45a2 , are associated with melanogenesis in vertebrates [3] , [51] , to the best of our knowledge, the others ( Ci-Mad/Mnt , Ci-Piwi , Ci-Lrp4 , Ci-Bzrap1 , Ci-Doc2a ) have not been implicated in pigmentation before. Interestingly, Ci-tyr , Ci-tyrp1/2a and Ci-tyrp1/2b are expressed in PCPs long before melanization begins [14] ( Fig. 10 ). This precocious expression of tyr in the pigment cell lineage is a feature shared with the vertebrates [15] . However, it is not clear why only the two posterior PCPs, a11.193 cell pairs, are finally melanized although all the cells express melanogenic genes. It has been suggested that this could be related to the differential tyr activity in the presumptive pigment cells, where it is finally lost in the most anterior PCP cells that do not become pigmented [52] . Additional melanocyte-specific constituents influence melanosome biogenesis, such as the availability of the tyr substrate, L -tyrosine, as well as the accumulation of the L -DOPA cofactor that governs its enzymatic activity. Perhaps the permeability of PCP cell membrane controls the time and rate of access of the tyr substrate and cofactor to the enzyme. Here, we showed that the expression of a subset of transcripts encoding membrane transporters (that is, Ci-Slc2a6 , Ci-Slc12a9 , Ci-Slc7a6 , Ci-Slc25a23 ) was decreased when FGF signalling was blocked in PCPs. In particular, Ci-Slc45a2 , the homologue of SLC45A2, which is responsible for oculocutaneous albinism type 4 in humans [51] , is selectively expressed in the posterior a11.193 cell pairs. These data suggest that FGF signalling could regulate melanization in the two posterior PCP cells by increasing the permeability and regulating the ionic composition of these cells. Here, we modelled a pigment cell lineage-specific transcriptional network to identify key effector genes involved in the early PCP induction and identified PCP-specific Ci-Rab32/38 as a hub gene. In mice, Rab32 and Rab38 control the trafficking of melanogenic enzymes (Tyr and Tyrp1) and are critical for melanosome maturation [40] . Moreover, it has been demonstrated that loss of Rab38 function alone causes a dramatic reduction in melanosome number within adult mouse RPE cells [43] . Also in Drosophila , mutation of Rab32/38 ortholog, Rab-RP1 , causes eye pigmentation defects [53] . These evidences parallel our finding in C. intestinalis where targeted perturbations of Ci-Rab32/38 activity interfere with a terminal melanization of the sensory organs. Considering the evolutionary relationship between the vertebrate small Rab GTPase members, Rab32 and Rab38, and the unique Ciona homologue, Ci-Rab32/38, ascidian pigment cells provide a simple and suitable system to identify the interacting partners for Rab32/38 and to study the functions of their regulators as well as the functional relationships with other factors during melanosome maturation. We showed that FGF signalling is involved in the early pigment cell type-specific regulation of several components of melanosome vesicular trafficking such as Ci-Rab32/38 and the melanophilin, Ci-Mlph , which are differential expressed in all pairwise comparisons at 8 hpf. Further studies are required to investigate the role of FGF signalling in the regulation of Ci-Rab32/38 and other melanosome-specific factors, thus offering insights on the molecular events underlying pigment cell biology. Furthermore, our microarray data revealed that FGF regulates the expression of known target-associated albinism or reduced pigmentation, such as HPS1 and LYST (Hermansky–Pudlak and Chédiak–Higashi syndromes [54] , [55] ). Therefore, it appears that Ciona pigment cells are endowed with the basic molecular machinery that underlies vertebrate melanosome biogenesis and that Ciona melanosomes may thus follow a biogenesis process similar to that observed in more complex organisms. In summary, the importance of Ci-Rab32/38 function during pigment cell formation together with the identification of Ci-Rab32/38 and Ci-Mlph as central hub genes in the inferred 8 hpf network, strongly suggest that FGF signalling regulates the expression of key effectors required to prime the molecular machinery for melanization since the early FGF-mediated induction on PCPs. Although detailed dissection of the different steps of Ciona melanosome maturation will require more in-depth analyses, Ciona pigmented cells provide an opportunity to analyse the conserved molecular basis of melanosome formation in vivo with high spatiotemporal resolution avoiding redundancy and compensations of vesicular trafficking components as well as the endocytic network that make difficult to dissect these cellular processes in a more complex system like vertebrates. Note added in proof : During correction of proof we found this paper related to our work. Nicolas Haupaix, Philip B. Abitua, Cathy Sirour, Hitoyoshi Yasuo,Michael Levine and Clare Hudson. (2014). Ephrin-mediated restrictionof ERK1/2 activity delimits the number of pigment cells in the /Ciona/CNS. Developmental Biology. In Press. PII: S0012-1606(14)00346-7; DOI: 10.1016/j.ydbio.2014.07.010. Animals and embryo electroporation Adult C. intestinalis were collected from the Gulf of Naples and, for microarray experiments, obtained from M-REP (San Diego, CA, USA). Ripe oocytes and sperm were collected surgically and kept separately until in vitro fertilization. We used a chemical dechorionation to eliminate chorion and follicular cells surrounding and protecting the eggs. Dechorionated eggs were then in vitro fertilized from different individuals. Fertilized eggs were washed in Millipore-filtered sea water (MFSW) transferred in a solution containing 0.77 M Mannitol and with the amount of DNA used for electroporation that was typically 50–80 μg of each plasmid. The electroporation was carried out in Bio-Rad Gene Pulser 0.4 cm cuvettes, using Gene Pulser II (Bio-Rad) [56] , [57] . Each experiment was performed at least three times. Embryos were staged according to the developmental timeline established in Hotta et al . [19] Embryo imaging capture was performed with a Zeiss Axio Imager M1 and a Zeiss LSM 510 META confocal microscope. Cell dissociation and FACS Embryonic cell suspensions for FACS were obtained as follows: stage-selected embryos were rinsed three times in artificial calcium and magnesium-free sea water (CMF-ASW: 449 mM NaCl, 33 mM Na2SO4, 9 mM KCl, 2.15 mM NaHCO3, 10 mM Tris-Cl pH 8.2, 2.5 mM EGTA) at room temperature. Embryos were dissociated by thorough pipetting for 2–3 min in 1 ml CMF-ASW supplemented with 0.1% trypsin (w/v, Sigma, T- 4799). Trypsin activity was blocked by adding ice-cold CMF-ASW supplemented with 0.1% bovine serum albumin (BSA, Sigma, A-3311). Cell suspensions were then rinsed three times with ice-cold CMF-ASW+BSA (cell were pelleted at 4 °C, by centrifugation at 3,000 r.p.m. (~500–700 g), for 2 min). Cell suspensions were maintained on ice and filtered into 5 ml polystyrene round bottom tubes equipped with a 40 μm cell-strainer cap (Falcon) before cell sorting [23] . Fluorescent-FACSof ptyrp1/2a>2xGFP and ptyrp1/2a>GFP-labelled PCP founder lineage cells was performed using, positive selection of GFP and negative selection of a MyoD905-driven Venus YFP on the FACS Aria (BD Bioscienes) sorter (New York University, Center for Genomics & Systems Biology). GFP and YFP fluorescence distributions were gated on the population of cells. Special attention was devoted to exclude debris and cell aggregates by gating. GFP fluorescence was collected using a 500 nm Dichroic long pass filter and a 510 nm discriminating optical filter. YFP fluorescence was collected using 550 nm Dichroic long pass filter and a 550 nm discriminating optical filter. For every sort, a non-fluorescent cell suspension as well as GFP-only and YFP-only samples were analysed to determine the optimal settings for sorting. Spectral overlap was adjusted using these samples to compensate for the GFP fluorescence component detected by the YFP detector and for the YFP fluorescence component detected by the GFP detector. Collimated GFP and YFP fluorescence was separated using 500 nm dichroic long pass filter. GFP fluorescence (fluorescence lower than 500 nm) was reflected towards a photomultiplier detector (PMT) with a 510 nm discriminating filter in front of it. YFP fluorescence was detected from the transmitted 500 nm dichroic long pass filter using a 550 nm dichroic long pass optical filter. A 550 nm discriminating optical filter was placed in the light path towards the designated YFP fluorescence PMT detector [23] . RNA Extraction and microarray hybridization The RNAqueous-Micro Kit (Ambion) was used for RNA extraction. RNA quality was assayed on Agilent Bioanalyzer 2100 with RNA 6000 Pico Chips and the associated kit (Agilent). RNA amplification and probe synthesis were performed using The Ovation Pico WTA System following manufacturer‘s recommendations (NuGen Technologies). The fragmented and labelled single-stranded cDNA targets were generated using the Encore Biotin Module (NuGen Techlonogies) following manufacturer’s recommendations (#4200-12). Hybridization to the C. intestinalis custom-design GeneChip was conducted using standard Affymetrix procedures (Affymetrix GeneChip Expression Analysis Technical Manual (P/N 702232 Rev. 2) at the New York University, Center for Genomics & Systems Biology. Microarray data analysis Affymetrix DAT files were converted into CEL files using proprietary software of the Affymetrix scanner. CEL files were loaded into the R statistical environment [58] (version 2.13.1) using the libraries Affy [59] and makecdfenv from the Bioconductor [60] collection of packages (version 2.8). The microarrays used in the present study represent an Affymetrix custom chip designed at the University of California, Berkeley and already used in gene expression studies of C. intestinalis [23] . Background correction, normalization and probe set summarization were performed using the Robust Multiarray Averaging method [61] with default parameters producing a single normalized expression value for each probe set in each sample. We first applied independent filtering of the expression measures to remove all the probe sets presenting low expression levels in all the samples or generally no expression variations. This increases the efficiency of the analysis by mitigating the effects of P value correction during the selection of differentially expressed genes [62] . Cut-offs for the independent filters were defined for each time point to maximize the number of significantly differentially expressed genes and were executed by performing the following comparisons at each time point: FGFR DN versus control, Ets:Vp16 versus control and FGFR DN versus Ets:Vp16. Expression values were analysed for differential expression using linear models and the empirical Bayes method from the Limma package [63] with default parameters. P values were adjusted using the Benjamini–Hochberg method [64] . We selected, as differentially expressed genes, only those genes associated to probe sets showing a corrected P value smaller than 0.1, which indicate a false discovery rate smaller than 10%. Microarray probe annotations and GO enrichment analyses Nucleotide sequences used to design the probes for each probe sets were obtained from the Affymetrix library file CINT06a520380F.sif. The next transcript models and annotations were downloaded from the ANISEED database [28] on March 2011: (1) JGI version 1, (2) KYOTOGRAIL2005, (3) KH and (4) ENSEMBL. ANISEED provides, for each transcript model sequence as well functional (homologues, GO, and so on) annotations. Transcript models and annotations were parsed and joined together to form a unique collection. Probe set sequences were then aligned against the collection of transcript models using BLAST+ (ref. 65 ) with the megablast algorithm option. Results were filtered to select exclusive hits with coverage >75% and identity >90%. Based on the selected hits, we associated each probe set to the corresponding transcript models and annotations. To perform such analysis, we developed custom Perl scripts that make extensive use of the BioPerl toolkit [66] . Finally, a MySQL database containing all the information downloaded and generated was used to collect and manage the data. GO functional enrichment analyses were performed using the collected GO annotations associated to the probe sets. We compared the GO classifications of specific subsets of probe sets (representing significantly differentially expressed transcripts and transcripts connected to hub genes) to the GO classifications of all the probe sets annotated on the whole microarray. For each GO class, we used the Fisher exact text and the P values were corrected using the Benjamini–Hochberg method. A summary table with the collected annotations and the code used in the analyses are publicly accessible at http://bit.ly/nPepdH . Reverse engineering of Ciona PCP co-regulatory network We computed the SCC for each pair of probes across the 24 microarrays, obtaining a correlation matrix of dimension 30,969 × 30,969. We estimated the SCC significance for each pair of probes by computing t statistics of each SCC value and then using a Student’s t -test distribution to estimate the P value. To control the number of false positives owing to the multiple hypotheses test problem, we estimated the degrees of freedom of the t -test distribution from the data by fitting the parameters of a Student’s t -location scale distribution to the t statistics computed for all the probe pairs. We estimated the parameters by minimizing the squared error between the theoretical and the empirical distribution. We also built a smaller early responsive to FGF signalling pathway subnetwork by starting from the top 50 differentially expressed transcripts (when comparing FGFR DN versus control at 8 hpf) and the transcripts connected to in the main network (gene neighbours). To identify ‘hub genes’ in this subnetwork, we ranked all the probe sets in the subnetwork according to their degree (that is, the number of connections a probe set has in the network). In situ hybridization The following ISH probes were obtained from plasmids contained in the C. intestinalis gene collection release I: tyrp1/2a (GC31h05), Bmp5/7 (GC46m03), Bzrap1(GC05h08), Doc2a (GC21m06), Lrp4 (GC42f11), Mad/Mnt (GC02d23), Rab32/38 (GC40p15), Six3/6 (GC11m13), FoxHa (GC32f03), Neurogenin (GC07n07), Pax3/7 (GC42e20), COE (GC02i14), Macho-1 (GC18g07), Msxb (GC42h24), Piwi (GC23f14) and full ORF Gateway-compatible clone: Casz1 (VES66_L10), RGR/Nut2 (VES94_E20), Pax6 (VES87_B20). PCR amplification of transcription templates was with the following oligos: Slc45a2 fw (5′-TCCCAGTGGGTATGATGTTG-3′) and Slc45a2 rev (5′-TTATTGGTTGCAGCACGAAG-3′). DIG- and FLUO-labelled probes were transcribed with T7 RNA polymerase (Roche) using DIG and FLUO labelling mix (Roche) and purified with the RNeasy Mini Kit (Qiagen). Single and double fluorescent ISH was performed as follows: Embryos were fixed at the different developmental stages for 2 h in 4% MEM-PFA (4% paraformaldehyde, 0.1 M MOPS pH 7.4, 0.5 M NaCl, 1 mM EGTA, 2 mM MgSO4, 0.05% Tween 20), then rinsed in cold phosphate-buffered saline (PBS) and stored in 75% ethanol at −20 °C. Before rehydration, embryos were treated with 2% H2O2 in methanol for 30 min at room temperature, and then rehydrated and manipulated as described through the post-hybridization washes. Embryos were then equilibrated in TNT (100 mM Tris pH 7.5, 150 mM NaCl, 0.1% Tween 20) and blocked in TNB (0.5% Roche blocking reagent in 100 mM Tris pH 7.5, 150 mM NaCl) for 1–2 h. Anti-FLUO-POD and anti-DIG-POD (Roche) antibodies were diluted 1:1,000 in TNB and incubated with embryos overnight at 4 °C. Embryos were washed extensively in TNT. For tyramide signal amplification, Cy3- and Cy5-coupled TSA Plus reagent (Perkin Elmer) was diluted 1:100 in amplification diluent and added to embryos for 5–10 min at room temperature. For 4,6-diamidino-2-phenylindole staining, DAPI (Sigma) was diluted 1:10,000 in PBT, and embryos were incubated overnight at 4 °C, then washed in PBT [67] . Embryo manipulation For antibody staining, embryos were fixed in 4% MEM-PFA for 30 min, rinsed several times in PBT (PBS with 0.1% Tween 20) and incubated with anti-dpERK antibody (Rabbit mAb, Cell Signalling technology, 1:100) and anti-GFP (Mouse mAb, Roche, 1:300) with 2% normal goat serum in PBT at 4 °C overnight. Embryos were washed in PBT and then incubated with donkey anti-mouse secondary antibody (1:500) coupled to Alexa Fluor 488 (Life Technologies) and anti-rabbit secondary antibody (1:500) coupled to Alexa Fluor 647 (Life Technologies) in PBT with 2% normal goat serum for 2 h at room temperature, then washed in PBT. For direct GFP and mCherry visualization, embryos were fixed in MEM-FA (3.7% methanol-free formaldehyde, 0.1 M MOPS pH 7.4, 0.5 M NaCl, 2 mM MgSO4, 1 mM EGTA) for 30 min, rinsed several times in PBS with 0.15% Triton X-100, 0.05% Tween 20 for 1 h. Drug treatments Embryos were obtained by in vitro fertilization, then chemically dechorionated and grown in MFSW at room temperature, until the desired stage. Experimental embryos were treated with 4 μM MEK inhibitor compound U0126 (Sigma) in MFSW (U0126 stock solution: 2 mM in dimethylsulphoxide) (Sigma) for 30 min and then washed with MFSW to remove the compound. Treated embryos were allowed to develop to the desired stage and then fixed for whole-mount ISH or immunohistochemistry. Construct preparation For cell sorting, PCPs were GFP labelled using ptyrp1/2a>2Xgfp (for 8 hpf) and ptyrp1/2a>GFP (for 12 hpf); the ptyrp1/2a minimal enhancer region is the same described in Esposito and coauthors [15] . For ptyrp1/2a>GFP, the GFP coding sequence was digested with XhoI and SmaI restriction enzymes and fused downstream from ptyrp1/2a promoter, replacing mCherry in the ptyrp1/2a>mCherry vector, previously digested with XhoI-EcoRV to eliminate mCherry. For ptyrp1/2a>2xGFP and ptyrp1/2a>LacZ, the tyrp1/2a enhancer was cloned upstream of the 2xGFP coding sequence and in the in the pBlueScript 1230 vector using NotI and EcoRI restriction sites. For ptyr>Rab32/38, the cDNA of Rab38/32 was amplified by PCR using as template the cDNA clone (N. Satoh Gene Collection 1 ID: CiGC40p15), with the oligonucleotides Rab32/38_Not FW (5′-AAGGAAAAAAGCGGCCGCTTTAATGACCGAACAAAGAAAGGA-3′) and Rab32/38_EcoRI REV (5′-CCGGAATTCCGGTTATCTGCAACAACCGCTCTTTTC-3′). Ci-Rab32/38 cDNA, digested with NotI/EcoRI was inserted in place of mCherry in the construct ptyrp1a>mCherry, previously digested with NotI-EcoRI to eliminate mCherry. Two different site-directed mutations in the GTPase domain of ptyr>Rab32/38 construct were induced to test Ci-Rab32/38 function. The first (ptyr>Rab32/38 G19V ) was prepared by a Gly to Val substitution in position 19 in the highly conserved phosphate/Mg 2+ domain, where GTP binding pocket is located. The second point mutation was a threonine to asparagine substitution in position 23 (ptyr>Rab32/38 G19V+T23N ), that disrupts the Mg 2+ binding site, resulting in greatly reduced affinity for guanine nucleotides. The point mutations were performed using (Quick Change Site-Directed Mutagenesis Kit from Stratagene/Agilent) using the following oligonucleotides: Rab32/38 G19V F (5′-gttcttgtgatcggcgagttagttgttgggaagacgagcgtcatt-3′), Rab32/38 G19V R (5′-aatgacgctcgtcttcccaacaactaactcgccgatcacaagaac-3′), Rab32/38 T23N F (5′-cgagttagttgttgggaagaatagcgtcattaaaagatat-3′), Rab32/38 T23N R (5′-atatcttttaatgacgctattcttcccaacaactaactcg-3′), shRNA-mediated RNA interference knockdown of Rab32/38 function The coding sequence of Ci- Rab32/38 was used to identify siRNA target sites with the DSIR [68] and Public TRC Portal ( http://www.broadinstitute.org/rnai/public/seq/search ) algorithms. Candidate 21-mer target sites were trimmed to 20 mer, and those that begin with A or G and end with A were further considered. Candidate 20 mer were BLASTed against the C. intestinalis genome on the Ghost database and selected to avoid polymorphic region as well as 20 mer with potential off-targets (that is, 16 nucleotide between positions 2 and 17 on the antisense). Target sense sequences were reverse complemented, and sense and antisense sequences were combined to mimic the hairpin structure corresponding to the microRNA miR-2213 (ref. 69 ). A vector containing the Ciona U6 promoter [70] was used to clone complementary oligos encoding four shRNA constructs: shRAB32/38-C-F 5′-agatGAAGAACGcgTTGGATAAttTGTAATTaGtAACATGTTATCCAAATCGTTCTTttt-3′ shRAB32/38-C-R 5′-aattaaaAAGAACGATTTGGATAACATGTTaCtAATTACAaaTTATCCAAcgCGTTCTTC-3′ shRAB32/38-D-F 5′-agatGAAGAACGcgTTGGATAAttTGTAATTaGtAACATGTTATCCAAATCGTTCTTttt-3′ shRAB32/38-D-R 5′-aattaaaAAGAACGATTTGGATAACATGTTaCtAATTACAaaTTATCCAAcgCGTTCTTC-3′ shRAB32/38-E-F 5′-agatGAAGAACGcgTTGGATAAttTGTAATTaGtAACATGTTATCCAAATCGTTCTTttt-3′ shRAB32/38-E-R 5′-aattaaaAAGAACGATTTGGATAACATGTTaCtAATTACAaaTTATCCAAcgCGTTCTTC-3′ shRAB32/38-F-F 5′-agatGAAGAACGcgTTGGATAAttTGTAATTaGtAACATGTTATCCAAATCGTTCTTttt-3′ shRAB32/38-F-R 5′-aattaaaAAGAACGATTTGGATAACATGTTaCtAATTACAaaTTATCCAAcgCGTTCTTC-3′ The data showed used 50 μg each of U6>shRab32/38-C, -D, -E, -F per electroporation. Accession codes : Microarray data are available in the ArrayExpress database ( www.ebi.ac.uk/arrayexpress ) under accession number E-MTAB-2759 . How to cite this article : Racioppi, C. et al. Fibroblast growth factor signalling controls nervous system patterning and pigment cell formation in Ciona intestinalis . Nat. Commun. 5:4830 doi: 10.1038/ncomms5830 (2014).